Tuning the band structure and superconductivity in single-layer FeSe by interface engineering The interface between transition metal compounds provides a rich playground for emergent phenomena. Recently, significantly enhanced superconductivity has been reported for single-layer FeSe on Nb-doped SrTiO 3 substrate. Yet it remains mysterious how the interface affects the superconductivity. Here we use in situ angle-resolved photoemission spectroscopy to investigate various FeSe-based heterostructures grown by molecular beam epitaxy, and uncover that electronic correlations and superconducting gap-closing temperature ( T g ) are tuned by interfacial effects. T g up to 75 K is observed in extremely tensile-strained single-layer FeSe on Nb-doped BaTiO 3 , which sets a record high pairing temperature for both Fe-based superconductor and monolayer-thick films, providing a promising prospect on realizing more cost-effective superconducting device. Moreover, our results exclude the direct correlation between superconductivity and tensile strain or the energy of an interfacial phonon mode, and highlight the critical and non-trivial role of FeSe/oxide interface on the high T g , which provides new clues for understanding its origin. The high-superconducting transition temperature ( T c ) in cuprate superconductors is hard to preserve in ultra-thin films as the monolayer limit approaches [1] . On the contrary, FeSe films grown on SrTiO 3 substrates show an enhanced T c with monolayer thickness [2] , [3] . Ex situ transport measurements of single-layer FeSe films (SLFs) grown on SrTiO 3 substrates (referred as FeSe S hereafter) with capping layers show an onset T c of ~40 K (ref. 4 ), much higher than the 8 K bulk value. Although the true T c of FeSe S remains to be confirmed by in situ transport measurements, in situ angle-resolved photoemission spectroscopy (ARPES) studies found a T g ~65 K (refs 5 , 6 ). This is the record high Cooper-pair-formation temperature among iron-based high-temperature superconductors (Fe-HTSs) and superconducting films at monolayer limit. It encourages further effort to increase T g above the liquid nitrogen boiling temperature, so that more cost-effective applications could be expected. One way is to explore different interfaces between FeSe and various oxides that would also provide more clues to understand the origin of the remarkable interfacial superconductivity in SLFs and high-temperature superconductivity in general. A burst of researches have been conducted recently on FeSe S , suggesting that the high T c might originate from epitaxial strain, interfacial electron–phonon coupling and/or charge transfer [6] , [7] , [8] , [9] , [10] . Here we directly manipulate these interfacial factors by heterostructure design. We have fabricated (1) SLFs with extremely expanded in-plane lattice of ~3.99 Å while preserving FeSe/SrTiO 3 interface by epitaxially growing FeSe/Nb:SrTiO 3 /KTaO 3 heterostructures (hereafter referred as FeSe SX ) [11] ; (2) SLFs with extremely expanded in-plane lattice of ~3.99 Å and with slightly expanded in-plane lattice of 3.78 Å, but changing the interfacial oxide to Nb-doped BaTiO 3 by epitaxially growing FeSe/Nb:BaTiO 3 /KTaO 3 heterostructures ( Fig. 1a , hereafter referred as FeSe B ); and (3) multi-layer Fe 1− x Co x Se films (hereafter referred as FeCoSe SR ), which are heavily electron doped similar to FeSe S but much thicker than SLFs. In situ ARPES studies were conducted on all these films to directly illustrate how the electronic structures and corresponding T g of FeSe films are affected by the interface. We demonstrate a record high Cooper-pair-formation temperature up to 75 K on FeSe B , extending the high-temperature superconductivity to new interfaces. Moreover, we found that the couplings between SLFs with the interfacial oxides renormalize the band structures in a non-trivial way. The band mass around the Brillouin zone centre is enhanced for SLFs with expanded lattice owing to the decrement of hopping terms, but the renormalization factor depends on the type of oxide substrate. On the other hand, the bandwidth of the electron-like bands around the Brillouin zone corners are negligibly affected. Furthermore, we exclude the direct relation between superconductivity and tensile strain, or the energy of an interfacial phonon mode, and demonstrate the crucial and non-trivial role of FeSe/oxide interface on the high T g . These results yield new microscopic insights into the high T c and provide clues for further enhancing T c through interface engineering. 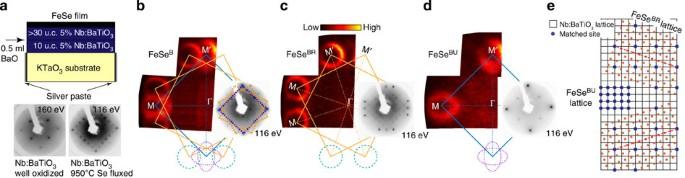Figure 1: The structures and Fermi surfaces of FeSe/Nb:BaTiO3/KTaO3films. (a) The schematic cross-section of the FeSe/Nb:BaTiO3/KTaO3films. For FeSeBU, 0.5 layer of BaO is inserted to eliminate the 3 × 3 superstructure as indicated. The LEED patterns for the Nb:BaTiO3/KTaO3films before and after the 950 °C heat treatment under Se flux are shown on the bottom. (b) Left: the Fermi surfaces of FeSeBas represented by the photoemission intensity map at the Fermi energy. The intensity was integrated over a window of (EF,EF−20 meV). Right: its LEED pattern. Besides the main spots that reflect the unrelaxed lattice of the substrate (indicated by the blue square), there are spots corresponding to two ±18.5° rotated lattices (indicated by the yellow squares). Correspondingly, there are three sets of Fermi surfaces whose respective Brillouin zone are derived based on the high symmetry points. (c) Left: the Fermi surfaces of FeSeBRresulting from post-annealing FeSeB, where only two sets of Fermi surfaces are observed, corresponding to the two ±18.5° rotated lattices. Right: its LEED pattern, where the main spots are weakened, and the spots for the rotated lattices are enhanced. (d) Left: the Fermi surfaces of FeSeBU, where only the elliptical Fermi surface sheets are observed. Right: its LEED pattern. No superstructure spots are observed and the lattice is unrelaxed. (e) Sketches for the lattices of various FeSe/Nb:BaTiO3/KTaO3films. Figure 1: The structures and Fermi surfaces of FeSe/Nb:BaTiO 3 /KTaO 3 films. ( a ) The schematic cross-section of the FeSe/Nb:BaTiO 3 /KTaO 3 films. For FeSe BU , 0.5 layer of BaO is inserted to eliminate the 3 × 3 superstructure as indicated. The LEED patterns for the Nb:BaTiO 3 /KTaO 3 films before and after the 950 °C heat treatment under Se flux are shown on the bottom. ( b ) Left: the Fermi surfaces of FeSe B as represented by the photoemission intensity map at the Fermi energy. The intensity was integrated over a window of ( E F , E F −20 meV). Right: its LEED pattern. Besides the main spots that reflect the unrelaxed lattice of the substrate (indicated by the blue square), there are spots corresponding to two ±18.5° rotated lattices (indicated by the yellow squares). Correspondingly, there are three sets of Fermi surfaces whose respective Brillouin zone are derived based on the high symmetry points. ( c ) Left: the Fermi surfaces of FeSe BR resulting from post-annealing FeSe B , where only two sets of Fermi surfaces are observed, corresponding to the two ±18.5° rotated lattices. Right: its LEED pattern, where the main spots are weakened, and the spots for the rotated lattices are enhanced. ( d ) Left: the Fermi surfaces of FeSe BU , where only the elliptical Fermi surface sheets are observed. Right: its LEED pattern. No superstructure spots are observed and the lattice is unrelaxed. ( e ) Sketches for the lattices of various FeSe/Nb:BaTiO 3 /KTaO 3 films. Full size image Two SLF domains of FeSe B with distinct in-plane lattices As shown by the in situ low-energy electron diffraction (LEED) patterns of the epitaxial Nb:BaTiO 3 ( Fig. 1a ), 3 × 3 surface reconstruction shows up after the heat treatment before SLF growth. From the photoemission spectral mapping and LEED image of FeSe B ( Fig. 1b ), we found that the reconstruction has a direct impact on the deposited SLFs by generating three spatially separated domains. One domain preserves the lattice of the KTaO 3 substrate, as highlighted by the blue square in the LEED pattern ( Fig. 1b ). The corresponding Fermi surfaces are elliptical ( Fig. 1b ), similar to those observed in FeSe SX (ref. 11 ). The other two domains are rotated about ±18.5°, as highlighted by the two yellow squares in the LEED pattern ( Fig. 1b ), and the corresponding Fermi surfaces consist of more circular sheets, similar to those observed in FeSe S . The in-plane lattice constant a of each domain could be derived from the inverted Brillouin zone size determined by high symmetry points of photoemission map [6] , which is 3.99 Å for the unrotated lattice and 3.78 Å for the rotated ones. As shown in Fig. 1e , these three domains of FeSe B match the reconstructed period. Particularly, every 10 periods of the rotated FeSe lattice match the diagonal of a 3 × 9 rectangle of the Nb:BaTiO 3 lattice (the dashed line in Fig. 1e ). Based on the calculated Luttinger volume, there are 0.12 excessive electrons per Fe for all these domains, similar to FeSe S and FeSe SX . The ±18.5° rotated domains could be further enhanced ( Fig. 1c ; such domains are referred as FeSe BR hereafter) with post annealing for over 15 h, while the unrelaxed domain could be enhanced ( Fig. 1d ; such a domain is referred as FeSe BU ) by insertion of extra BaO layer in Nb:BaTiO 3 film ( Fig. 1a ). In this way, the electronic structures and corresponding T g can be compared in different domains of FeSe B with the lattice constant as a clean control parameter. Interface-induced band structure evolution In Fig. 2 , we present the band dispersions for various SLFs grown on Nb:BaTiO 3 or Nb:SrTiO 3 . Around Γ(0,0), the generic features for all films include a parabolic band α and a relative flat band ω at higher binding energy ( Fig. 2a,b ). Since the bands around zone centre are nearly isotropic, the photoemission cuts with different in-plane angles are comparable ( Supplementary Fig. 1 ). For the two films grown on Nb:BaTiO 3 , the larger a corresponds to a larger effective mass of band α and smaller energy separations between the two bands ( Fig. 2b(i,ii) ). The same holds true for the two SLFs grown on Nb:SrTiO 3 ( Fig. 2b(iii,iv) ). Density functional theory (DFT) calculations were performed for FeSe SX and FeSe S , showing that the band mass and band separation indeed increases with the expanded lattice ( Fig. 2c(ii,iii) ), similar to the experimental results. Quantitatively, we scale the measured bands to the calculated ones, and get the same renormalization factor of 5.0 for both FeSe SX ( Fig. 2c(ii) ) and FeSe S ( Fig. 2c(iii) ). Therefore, the quasiparticle bandwidth narrowing with enhanced tensile strain could be fully attributed to a pure band effect, that is, the decrement of the hopping integral t . Consequently for such an iron-based superconductor, the electronic correlation strength is enhanced with the expanded lattice, since it could be represented by either J H / t (refs 12 , 13 ) or J 2 / t (ref. 14 ; J H being the on-site Hund’s rule coupling constant, and J 2 being the next-nearest-neighbour exchange coupling parameter). 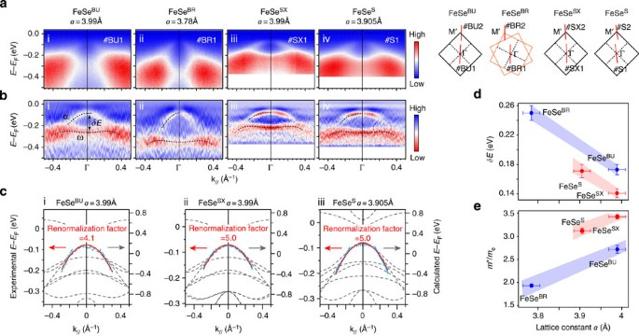Figure 2: The band structures around the zone centre of various FeSe films. (a,b) The photoemission intensity along #BU1, #BR1, #SX1 and #S1 across Г (a(i–iv)), and the corresponding second derivative with respect to energy to highlight the dispersions (b(i–iv)) for FeSeBU, FeSeBR, FeSeSXand FeSeS, respectively. The momentum location of the cuts are shown in the top-right inset. (c) Comparison of the dispersion of band α from ARPES data and the DFT calculated band structures along the Г-M′ direction. The blue markers show the experimental dispersions and the red curves show the corresponding parabolic fittings. The energy scales of the calculated band structures at the right side are several times of the energy scales of the experimental data at the left, and the corresponding renormalization factors are shown. The #BU1 and #BR1 data were taken at 45 K, whereas others were taken at 30 K. (d) The energy separations between the α and ω bands at Г versus . The energy separation is defined inb(i). (e) Effective massm* of band α as a function of in-plane lattice constant , wheremeis the free-electron mass. The effective mass is determined by parabolic fitting of the band dispersion of band α. The error bars for band separation and effective mass are determined by the combination of energy resolution, fitting errors and deviations between samples. The error bar for is owing to the uncertainty in determining the Brillouin zone size from features with finite width. We note that the slight rotation of the cuts does not affect the quantitative conclusions here (Supplementary Fig. 1). Figure 2: The band structures around the zone centre of various FeSe films. ( a , b ) The photoemission intensity along #BU1, #BR1, #SX1 and #S1 across Г ( a (i–iv)), and the corresponding second derivative with respect to energy to highlight the dispersions ( b (i–iv)) for FeSe BU , FeSe BR , FeSe SX and FeSe S , respectively. The momentum location of the cuts are shown in the top-right inset. ( c ) Comparison of the dispersion of band α from ARPES data and the DFT calculated band structures along the Г-M′ direction. The blue markers show the experimental dispersions and the red curves show the corresponding parabolic fittings. The energy scales of the calculated band structures at the right side are several times of the energy scales of the experimental data at the left, and the corresponding renormalization factors are shown. The #BU1 and #BR1 data were taken at 45 K, whereas others were taken at 30 K. ( d ) The energy separations between the α and ω bands at Г versus . The energy separation is defined in b (i). ( e ) Effective mass m * of band α as a function of in-plane lattice constant , where m e is the free-electron mass. The effective mass is determined by parabolic fitting of the band dispersion of band α. The error bars for band separation and effective mass are determined by the combination of energy resolution, fitting errors and deviations between samples. The error bar for is owing to the uncertainty in determining the Brillouin zone size from features with finite width. We note that the slight rotation of the cuts does not affect the quantitative conclusions here ( Supplementary Fig. 1 ). Full size image Intriguingly, even though both the Nb:BaTiO 3 /KTaO 3 and Nb:SrTiO 3 /KTaO 3 provide similar amount of electrons to SLFs and poss the same tensile strain with a =3.99 Å, there are clear differences in the band dispersions for FeSe SX and FeSe BU ( Fig. 2b(i,iii) ). The bands are flatter for SLFs on Nb:SrTiO 3 than that for SLFs on Nb:BaTiO 3 . However, in our DFT calculations, the calculated band structure for FeSe BU is similar to that of FeSe SX ( Fig. 2c(i,ii) ), which could not account for the band mass variation with different interfacial oxides as observed in our experiments ( Fig. 2b(i,iii) ). The renormalization factor between the measured α band and the calculated one is 4.3 for FeSe BU ( Fig. 2c(i) ), which is smaller than that of FeSe SX ( Fig. 2c(ii) ). Therefore, the bandwidth variations for SLFs on different oxides are beyond the pure lattice-expansion effect, and there should be additional correlation effects that depend on the interface. As summarized in Fig. 2d,e , the two characteristic quantities (band mass and band separation) fall on two separate curves as a function of a , which clearly indicates that the interfacial oxide material has non-trivial effects on the electronic correlation of the epitaxial SLFs. The different interfacial oxides and strains affect the band structure around M ( π ,0) as well, but in a different non-trivial manner ( Fig. 3a,b ). For FeSe BR and FeSe S with smaller in-plane lattices, the two γ1 and γ2 bands are degenerating ( Fig. 3b(ii,iv) ). For the large a =3.99 Å, two γ1 and γ2 electron bands are resolved for FeSe BU and FeSe SX but with different separations between them ( Fig. 3b(i,iii) ). Remarkably, unlike the different renormalizations of the α band, the bandwidths of the electron bands are similar in all these films. 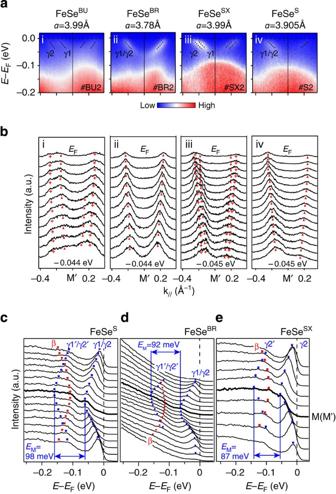Figure 3: The band structures around the zone corner of various FeSe films. (a,b) The photoemission intensity along #BU2, #BR2, #SX2 and #S2 across M′ (a(i–iv)), and the corresponding momentum distribution curves (b(i–iv)) for FeSeBU, FeSeBR, FeSeSXand FeSeS, respectively. The momentum locations are illustrated in the top-right inset ofFig. 2. (c–e) Energy distribution curves (EDCs) across M(M′) for FeSeS, FeSeBRand FeSeSX, respectively, which show band replication behaviour. The markers are local maximum locus to indicate the band position, and the replica bands are labelled as γ1′/γ2′ or γ2′ considering the band degeneracy and matrix element effects11. The energy separations between the main band and the replica band are shown asEMfor different SLFs to represent the energy scales of the phonon modes. The data were taken at 30 K. Figure 3: The band structures around the zone corner of various FeSe films. ( a , b ) The photoemission intensity along #BU2, #BR2, #SX2 and #S2 across M′ ( a (i–iv)), and the corresponding momentum distribution curves ( b (i–iv)) for FeSe BU , FeSe BR , FeSe SX and FeSe S , respectively. The momentum locations are illustrated in the top-right inset of Fig. 2 . ( c – e ) Energy distribution curves (EDCs) across M(M′) for FeSe S , FeSe BR and FeSe SX , respectively, which show band replication behaviour. The markers are local maximum locus to indicate the band position, and the replica bands are labelled as γ1′/γ2′ or γ2′ considering the band degeneracy and matrix element effects [11] . The energy separations between the main band and the replica band are shown as E M for different SLFs to represent the energy scales of the phonon modes. The data were taken at 30 K. Full size image Replica bands near M and interfacial phonon energy scale At higher binding energies, replicas of the electron bands (those of γ1 and/or γ2 bands considering the band degeneracy and matrix element effects [11] ) can be resolved in FeSe S , FeSe BR and FeSe SX ( Fig. 3c–e ) near M. Such band replication behaviour was observed in FeSe S , which has been shown to be very likely a shake-off satellite band by an interfaical oxygen optical phonon mode [10] . In ref. 10 , a sophisticated spectral lineshape fitting was exploited to retrieve the energy of this phonon, and its coupling strength to the electrons. However, since the intensity ratio between the replica bands and the corresponding main bands are influenced by the photoemission matrix element effect and sample quality, we could not directly extract the coupling strengths at different interfaces from our data. Nevertheless, one could take the energy separation between the main band and the replica band to represent the energy scale of the phonon mode, E M , which is 98, 92 and 87 meV for FeSe S , FeSe BR , and FeSe SX , respectively ( Fig. 3c–e ). Cooper-pair-formation temperature The superconducting properties of the various SLFs are examined in Fig. 4 . 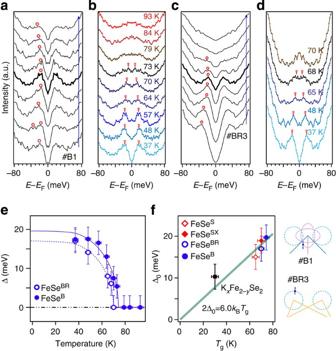Figure 4: Temperature dependence of the superconducting gaps for different FeSe films. (a) The symmetrized EDCs for FeSeBalong cut #B1 as indicated in the bottom-right inset. The circles mark the dispersion. The thick EDC curve is at the normal state Fermi momentum (kF) of the FeSeBUdomain. (b) Temperature dependence of the symmetrized EDC at the markedkFfor FeSeB. The coherent peak positions are marked by triangles. (c,d) Similar asa,b, but for FeSeBRfilm. (e) The superconducting gap determined as a function of temperature from data inb,d. The solid and dashed curves are the fits by the Bardeen–CooperSchrieffer gap-temperature formula. (f) The maximal low-temperature gap versusTgplot, including the values for KxFe2−ySe2bulk31, FeSeS(ref.6) and FeSeSX(ref.11). Note that for FeSeSXand FeSeB, the maximal values of the anisotropic gap distributions are used. The error bars of temperature are from the measurement uncertainty, and those of gap are from the s.d. of the fitting process. Figure 4a shows the symmetrized energy distribution curves (EDCs) at low temperature along cut #B1 across the Fermi surfaces of the unrotated domains of FeSe B . The dispersion exhibits a characteristic bending back behaviour after passing the Fermi momentum. This is a hallmark of Bogliubov quasiparticle dispersion, and indicates that the gap is due to Cooper-pair formation. The gap amplitude of FeSe B shows anisotropic distribution along the elliptical Fermi surfaces of the unrotated domain ( Supplementary Fig. 2 ), which is consistent with our previous results on FeSe SX (ref. 11 ). The symmetrized EDCs at the normal state Fermi momenta could be used to identify the gap by the spectral weight suppression at E F , which is minimally affected by the temperature broadening effects [15] . Figure 4b presents the temperature dependence of the symmetrized EDCs at the Fermi momentum for the unrotated domains in FeSe B , and the gap decreases with increasing temperature and eventually closes above 73 K. In Fig. 4c,d , we show the gap behaviour of FeSe BR , and the gap closes above 68 K. The data for FeSe BU shows rather weak coherence peaks, but with possible signs for T g above 77 K ( Supplementary Fig. 3 ). Figure 4: Temperature dependence of the superconducting gaps for different FeSe films. ( a ) The symmetrized EDCs for FeSe B along cut #B1 as indicated in the bottom-right inset. The circles mark the dispersion. The thick EDC curve is at the normal state Fermi momentum ( k F ) of the FeSe BU domain. ( b ) Temperature dependence of the symmetrized EDC at the marked k F for FeSe B . The coherent peak positions are marked by triangles. ( c , d ) Similar as a , b , but for FeSe BR film. ( e ) The superconducting gap determined as a function of temperature from data in b , d . The solid and dashed curves are the fits by the Bardeen–CooperSchrieffer gap-temperature formula. ( f ) The maximal low-temperature gap versus T g plot, including the values for K x Fe 2− y Se 2 bulk [31] , FeSe S (ref. 6 ) and FeSe SX (ref. 11 ). Note that for FeSe SX and FeSe B , the maximal values of the anisotropic gap distributions are used. The error bars of temperature are from the measurement uncertainty, and those of gap are from the s.d. of the fitting process. Full size image The temperature dependence of the gap is shown in Fig. 4e , which could be well fitted by the Bardeen–CooperSchrieffer gap versus temperature formula. This further suggest that the gap-opening relates to the Cooper-pair formation, although in situ transport is needed to check if T c = T g . The fitted T g is 75±2 K, and 70±2 K for FeSe B and FeSe BR , respectively. The former sets a record high T g for Fe-HTSs and monolayer-thick films. Figure 4f summarizes the maximal gap versus T g for FeSe films and K x Fe 2− y Se 2 . One can find a monotonic and generally linear trend between T g and the gap amplitude, with 2Δ/ k B T c ~6.0, demonstrating the relatively strong coupling superconductivity and the similar superconducting nature in these materials. Crucial role of FeSe/oxide interface on the high T g Considering that high T g seems robust in all these SLFs, especially in FeSe BR whose a is close to that of bulk FeSe (3.765 Å), it is intriguing to check whether thick FeSe films with the same a and similar electron doping of FeSe BR would also hold high T g . We have grown 35-unit cell (u.c. )-thick FeCoSe SR on Nb:SrTiO 3 with the electron carriers introduced by Co doping, and its a is relaxed to 3.78 Å as derived from the inversed Brillouin zone size [6] . As shown in Fig. 5a,b , the hole pockets formed by bands α and β sink below the Fermi energy, and the electron Fermi surfaces are fairly large as shown in Fig. 5c–e . About 8% electrons could be doped, which is limited by the solubility of cobalt. The symmetrized EDCs at 30 K across the electron Fermi surfaces are shown in Fig. 5f,g , however, without any sign of a superconducting gap. The T g , if any, is below the lowest temperature of 30 K that could be reached at the current experimental setup. If the superconductivity had been originated only from the FeSe layer, one would expect a higer T g in FeCoSe SR owing to suppressed two-dimensional (2D) fluctuations in thick films, which is not observed in our experiments. This demonstrates the dominating role of the FeSe/oxide interface on the high T g in FeSe/Nb:SrTiO 3 or FeSe/Nb:BaTiO 3 . In thick FeCoSe SR films where interfacial effects are negligible, the absence of a gap or a small T g is expected, since heavy electron doping would bring the system to the overdoped regime, where superconductivity diminishes as observed for bulk Fe-HTSs [16] , [17] . 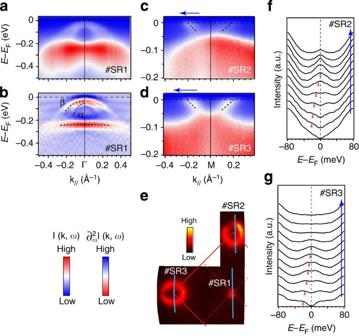Figure 5: Electronic structure of FeCoSeSR. FeCoSeSRis a Co-doped 35-u.c.-thick FeSe film with partially relaxed lattice. (a,b) The photoemission intensity (a) and the corresponding second derivative with respect to energy to highlight the dispersions (b) along cut #SR1. (c,d) The photoemission intensity along cut #SR2 and cut #SR3, respectively. (e) Photoemission intensity map atEFfor FeCoSeSR, which is integrated over (EF+10 meV,EF−10 meV), where the momentum cuts for data in other panels are marked. (f,g) The symmetrized EDCs along a portion of cut #SR2 (f) and cut #SR3 (g), as indicated by the blue arrows inc,d, respectively. The dispersions are marked by the red triangles. The data were taken at 30 K. Figure 5: Electronic structure of FeCoSe SR . FeCoSe SR is a Co-doped 35-u.c.-thick FeSe film with partially relaxed lattice. ( a , b ) The photoemission intensity ( a ) and the corresponding second derivative with respect to energy to highlight the dispersions ( b ) along cut #SR1. ( c , d ) The photoemission intensity along cut #SR2 and cut #SR3, respectively. ( e ) Photoemission intensity map at E F for FeCoSe SR , which is integrated over ( E F +10 meV, E F −10 meV), where the momentum cuts for data in other panels are marked. ( f , g ) The symmetrized EDCs along a portion of cut #SR2 ( f ) and cut #SR3 ( g ), as indicated by the blue arrows in c , d , respectively. The dispersions are marked by the red triangles. The data were taken at 30 K. Full size image Our results help to illucidate and/or exclude some of the interfacial effects on the superconductivity in SLFs. Particularly, the interfacial tensile strain has been proposed to be a critical factor [6] that normally would significantly enhance the antiferromagnetic superexchange interactions across the Fe-Se-Fe [8] . However, with the lattice expansion by 5.5% in FeSe BU compared with FeSe BR , T g is enhanced by only 5 K ( Fig. 6a ), surprisingly small in the context of the antiferromagnetic-interaction/spin fluctuations-mediated superconductivity, which is arguably the current dominating picture for bulk Fe-HTSs [18] . The lattice expansion from FeSe S to FeSe SX induces small T g enhancement as well [11] . Therefore, the tensile strain imposed by the oxide layer is a positive but not a major factor for the high T g in SLFs. In addition, as shown in Fig. 6a , the large T g enhancement from FeCoSe SR to FeSe BR is due to interfacial effects beyond tensile strain, since they have the same in-plane lattice. 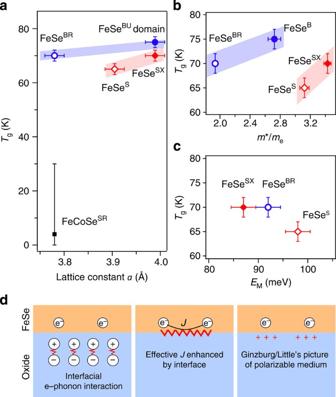Figure 6: The relation betweenTgand various parameters. (a)Tgas a function of in-plane lattice constanta. TheTgof FeCoSeSRis below the lowest temperature of 30 K that could be reached at the current apparatus. Since FeCoSeSRis overdoped with essentially no interface effects, itsTgshould be lower than the bulk FeSeTcof 8 K, assuming that it possesses the common superconducting dome of Fe-HTSs. Here we expect itsTgat 4 K, with the error bar between 0 and 30 K. The other error bars ofTgare from the measurement uncertainty, and those ofaare owing to the uncertainty in determining the Brillouin zone size from features with finite width. (b)Tgas a function of the effective mass of band α at the zone centre. The error bars of effective mass are determined by the combination of energy resolution and fitting errors. (c)Tgversus the energy scale of the phonon mode represented asEM. The error bars ofEMare determined from the experimental resolution. (d) Illustration of three possible paring mechanisms for the highTgin SLFs. Figure 6: The relation between T g and various parameters. ( a ) T g as a function of in-plane lattice constant a . The T g of FeCoSe SR is below the lowest temperature of 30 K that could be reached at the current apparatus. Since FeCoSe SR is overdoped with essentially no interface effects, its T g should be lower than the bulk FeSe T c of 8 K, assuming that it possesses the common superconducting dome of Fe-HTSs. Here we expect its T g at 4 K, with the error bar between 0 and 30 K. The other error bars of T g are from the measurement uncertainty, and those of a are owing to the uncertainty in determining the Brillouin zone size from features with finite width. ( b ) T g as a function of the effective mass of band α at the zone centre. The error bars of effective mass are determined by the combination of energy resolution and fitting errors. ( c ) T g versus the energy scale of the phonon mode represented as E M . The error bars of E M are determined from the experimental resolution. ( d ) Illustration of three possible paring mechanisms for the high T g in SLFs. Full size image The correlation between T g and the complex interfacial effects on the band renormalizations around Γ and M deserves further examination. The correlation strength deduced from the α band varies with different interfacial oxides and tensile strain, as indicated by the effective mass in Fig. 2e . However, as shown in Fig. 6b , T g does not monotonically correlate with the quasiparticle mass of the α band. This is not surprising as α is fully occupied and does not contribute to pairing. Intriguingly, for the partially occupied electron-like bands around M that contribute to pairing, their band bottoms are all around −60 meV for the same doping of 0.12e − per Fe in different SLFs ( Fig. 3 ), giving almost identical bandwidth for the electron bands in these SLFs, although their Fermi velocities could not be directly compared owing to the different band degeneracies. The nearly same bandwidth for the partially occupied electron bands may relate to the robust high-superconducting gap-closing temperatures in these SLFs [19] . With the above observations, one could speculate some intriguing and non-exclusive possibilities as illustrated in Fig. 6d . For example, the polarizability of the ions in the oxide layer induces interfacial electron–phonon interactions [20] . Consistenly, we have observed the general presence of the related replica band ( Fig. 3c–e ) at the SLF/oxide interfaces. The high-frequency phonons and strong electron–phonon interactions in Nb:SrTiO 3 or Nb:BaTiO 3 may mediate superconductivity as proposed in ref. 9 . However, Fig. 6c clearly rules out the direct correlation between E M and T g . Further direct evidence is required to see whether the electron–phonon coupling strength or the combination of the coupling strength and phonon energy would correlate with T g . Another possibility is that the pairing is mediated by certain antiferromagnetic interaction J in SLFs, which sets the scales of both the superconducting gap and T g . If so, our results demonstrate that there is a non-trivial enhancement from the FeSe/oxide interface to J , which is beyond the simple tensile strain effects, and may be manifested in the relatively unchanged bandwidth of the electron-like band around M. In addition, we did not find any noticeable dependence of the electronic structure and superconducting properties on the Nb concentration (that is, conductivity and carrier density in the oxide layer). Therefore, it is not likely that the superconductivity in SLFs is mediated by the electronic polarizability of the substrate following the picture proposed by Little [21] and Ginzburg [22] . Nevertheless, the electronic polarizability of the substrate would help to screen the Coulomb interactions at various ranges [23] , thus facilitate pairing [24] . In fact, the observed interfacial oxide dependence of correlations in SLFs may be resulting from the different screening of the interactions by Nb:SrTiO 3 and Nb:BaTiO 3 . Thin film growth Before oxide thin film growth, (001) oriented KTaO 3 substrates were etched with buffered NH 4 -HF solutions and annealed in 2 bar pure oxygen to get atomically smooth surface. Oxide thin films (including 5% Nb-doped BaTiO 3 films, 5% Nb-doped SrTiO 3 films and 0.5% Nb-doped SrTiO 3 films) were grown with ozone-assisted molecular beam epitaxy following the shutter-controlled layer-by-layer growth method: the A site material (Ba or Sr) and B site materials (Ti and Nb) were deposited alternatively, while Ti and Nb were co-deposited to get uniform doping [25] . The relative stoichiometry and absolute amount of each element were based on quartz crystal microbalance measurements and the real-time reflection high-energy electron diffraction oscillation method described in ref. 25 . During the growth of oxides, the reflection high-energy electron diffraction pattern retained its 2D character. With the shutter-controlled growth mode [25] , the films were terminated with TiO 2 layer after the growth of each unit cell. The oxide films were typically 40-u.c. thick. Nb doping is induced, and silver paste was attached on the substrate edge in order to improve the conduction of oxide layer and avoid charging effect during photoemission measurements. After the growth of oxides, the heterostructures were transferred under an ultra-high vacuum to another molecular beam epitaxy (MBE) chamber, where they were heated to 950 °C with Se flux for 30 min. FeSe films were co-deposited with the Se flux 20 times greater than the Fe flux while the substrates were kept at 450 °C. FeCoSe SR films were grown directly on TiO 2 -terminated Nb:SrTiO 3 substrates with 8% amount of Fe substituted by Co. Afterwards, the films were annealed at 600 °C in vacuum for 3 h and directly transferred into the ARPES chamber. Longer annealing increases the relaxed domain (FeSe BR ) in FeSe B and improves film quality in most cases, while it does not notably change the band structure. ARPES measurement ARPES data were taken in situ under ultra-high vacuum of 1.5 × 10 −11 mbar, with a SPECS UVLS discharge lamp (21.2 eV He-Iα light) and a Scienta R4000 electron analyser. The energy resolution is 8 meV and the angular resolution is 0.3°. Data were taken at 30 K if not specified otherwise. To eliminate the photoemission charging effect due to insulating KTaO 3 , silver paste was attached on the substrate edge before growth. First-principles calculations To study the electronic structure of FeSe monolayers, we used the first-principles calculations by the projector augmented wave method [26] implemented in Vienna Ab-initio Simulation Package (VASP) package [27] , [28] . We adopted the generalized gradient approximation of Perdew–Burke–Ernzerhof for the exchange–correlation potentials [29] . The kinetic energy cutoff of the plane-wave basis was set to be 400 eV after the full convergence test. The optimization made the forces on all relaxed atoms smaller than 0.01 eV/Å. To model the band structure of FeSe monolayer on top of TiO 2 -terminated SrTiO 3 (001), a six-layer SrTiO 3 (001) slab was used with the FeSe monolayer adsorbed on the top side in a a × a 2D u.c. plus a vacuum layer of 10 Å, while setting the lattice parameters to a =3.905 and 3.989 Å for FeSe S and FeSe SX , respectively. The top two slab layers and all FeSe layer atoms were allowed to relax, whereas other slab layers were fixed at at their original positions. A 12 × 12 k -points mesh for the Brillouin zone sampling and a width of 0.1 eV Gaussian smearing were used. The electric field induced by asymmetric atomic relaxation was compensated by a dipole correction [30] . To model FeSe BU , same method was used except changing the six-layer SrTiO 3 (001) slab to six-layer BaTiO 3 (001) slab. Owing to its large unit cell, we were not able to calculate the band structure of FeSe BR . How to cite this article : Peng, R. et al . Tuning the band structure and superconductivity in single-layer FeSe by interface engineering. Nat. Commun. 5:5044 doi: 10.1038/ncomms6044 (2014).